Global potential of biospheric carbon management for climate mitigation Potential pathways to climate stabilization require the deployment of a broad portfolio of solutions to increase energy efficiency, replace fossil fuel use and remove GHGs. The technological solutions available to address these challenges can be broadly divided into two camps: (1) non-biological solutions that do not involve the biosphere, such as wind and solar farms for the generation of electricity and (2) biological solutions that do involve biospheric components of the natural and managed carbon cycle, such as bioenergy or reforestation. Biological solutions are distinctive in at least two ways. First, large terrestrial and ocean carbon sinks (reservoirs that accumulate and store carbon) already exist and remove more than half of the annual anthropogenic CO 2 emissions from the atmosphere [1] , [2] . Thus, understanding and management of the dynamics of these sinks is of paramount importance. Second, most biological mitigation activities require additional harvesting of the Earth’s plant production (that is, net primary production) beyond its current 38% use [3] . However, these requirements face the limitation that a third of the terrestrial plant production is belowground, which is not economically harvestable, and another third takes place on difficult or remote terrain. Thus, there is a clear natural limit to the global fraction further available for human exploitation. Only 10% of the land surface, equivalent to 5 PgC per year (petagrams of carbon per year=10 15 g=a billion metric tonne) [3] , remains. There is a need to exploit a larger fraction of biomass production for the purpose of climate change mitigation that would place this goal in direct competition with the agendas of food security, energy security and often biodiversity conservation [4] , all of which also require increasing quantities of biomass and land to meet their goals ( Fig. 1 ). In addition, an emerging bio-economy intending to replace many of the petroleum-based products by plant-based products [5] , [6] will put further demands on biomass production. 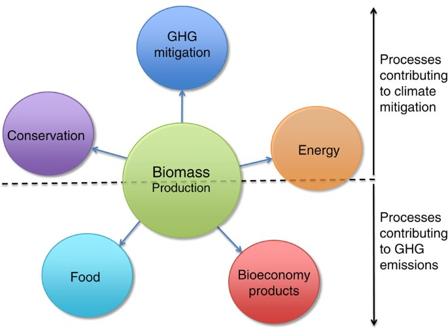Figure 1: Demands on biomass from multiple sectors. Biomass applications that can directly contribute to climate mitigation are conservation (for example, reduced deforestation with other benefits on the provision of ecosystem services), GHG mitigation (for example, reforestation) and energy (for example, bioenergy production when replacing fossil fuels). The production of food and products for an emerging bio-economy is a net source of GHGs. Figure 1: Demands on biomass from multiple sectors. Biomass applications that can directly contribute to climate mitigation are conservation (for example, reduced deforestation with other benefits on the provision of ecosystem services), GHG mitigation (for example, reforestation) and energy (for example, bioenergy production when replacing fossil fuels). The production of food and products for an emerging bio-economy is a net source of GHGs. Full size image New technologies will contribute to improving the sustainable production and conversion of biomass for a range of food, fibre, energy, health and industrial products. However, with new demands, there will also be unprecedented challenges as a larger economy is created on the increasingly valuable biomass commodity, which is further confronted by the unfolding of climate change. Ultimately, the concept of sustainable development must govern any further intensification of the biosphere that is consistent with the original United Nations’ definition ‘Development that meets the needs of the present without compromising the ability of future generations to meet their own needs’ [7] . In this review article, we assess the potential of a number of currently available land-based biological carbon mitigation activities that can be achieved with a high degree of environmental sustainability by 2050. We place this potential in the context of the requirements for large-scale deployment of mitigation activities, the dynamics of the carbon cycle and the mitigation requirements for climate stabilization. We also discuss new frontiers in research and development (R&D) on technologies that, if successful, would decrease the demands on land and biomass. We conclude that, for now and in the coming decades, continuous intensification of land use with a high degree of sustainability, while realising the opportunity to enable limited, but significant, land-based mitigation in the form of avoided emissions from deforestation and agriculture and production of bioenergy, remains the biggest challenge. The global carbon cycle is being perturbed by emissions from the combustion of fossil fuels and by changes in land use and land-use intensity. These perturbations have led to cumulative anthropogenic CO 2 emissions of 570±70 PgC since the beginning of the Industrial Era (1750) to 2012. Seventy percent (385±20 PgC) of these emissions originated from the combustion of fossil fuels and 30% (185±65 PgC) from land use (for example, intensification of plant production) and from land-use change (for example, deforestation and reforestation) [2] . For the most recent decade (2003–2012), land-use change was responsible for 10% of total anthropogenic carbon emissions ( Fig. 2 ; Table 1 ). 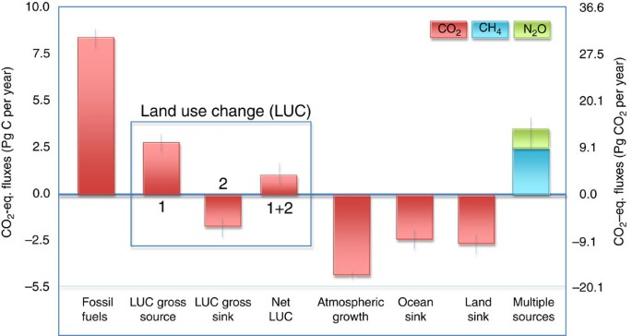Figure 2: Fluxes of GHGs associated with human activities. CO2for the period 2003–2012 based on refs1,2,13,77, and CH4and N2O25,78for the 2000s (as inTable 1). The left vertical axis shows units in PgC per year for the three gases (CH4and N2O calculated from CO2-eq) and the right vertical axis shows units in PgCO2-eq per year for the three gases. The land-use change (LUC) box shows the two gross fluxes: (1) emissions to the atmosphere from deforestation and (2) removal from the atmosphere by regrowth and reforestation/afforestation), which make the net flux to the atmosphere (1+2)13. For CO2(red), bars show the complete mass balance budget of anthropogenic emissions to the atmosphere (positive values) and sinks to land and oceans (negative values). For CH4and N2O (blue and green, respectively), only anthropogenic emissions are shown for comparison with CO2emissions. Figure 2: Fluxes of GHGs associated with human activities. CO 2 for the period 2003–2012 based on refs 1 , 2 , 13 , 77 , and CH 4 and N 2 O [25] , [78] for the 2000s (as in Table 1 ). The left vertical axis shows units in PgC per year for the three gases (CH 4 and N 2 O calculated from CO 2 -eq) and the right vertical axis shows units in PgCO 2 -eq per year for the three gases. The land-use change (LUC) box shows the two gross fluxes: (1) emissions to the atmosphere from deforestation and (2) removal from the atmosphere by regrowth and reforestation/afforestation), which make the net flux to the atmosphere (1+2) [13] . For CO 2 (red), bars show the complete mass balance budget of anthropogenic emissions to the atmosphere (positive values) and sinks to land and oceans (negative values). For CH 4 and N 2 O (blue and green, respectively), only anthropogenic emissions are shown for comparison with CO 2 emissions. Full size image Table 1 Global annual mean fluxes of greenhouse gases. Full size table The accumulation of excess atmospheric CO 2 and increases in nitrogen (N) deposition have resulted in a physical and biological response in the form of the creation of natural carbon sinks. Of the historical cumulative emissions of 570±70 PgC between 1750 and 2012, the ocean and land carbon sinks have removed 165±20 and 160±70 PgC, respectively, with 245±5 PgC remaining in the atmosphere [2] . Although CO 2 is the most abundant and important well-mixed GHG, other gases, mainly methane (CH 4 ) and nitrous oxide (N 2 O), also contribute to human-induced climate change. Here we use the CO 2 -equivalent (eq) metric to compare the three gases, which is the amount of CO 2 that would have the same global warming potential as another gas over a given time period (100 years used here). On the basis of the global warming potential of CO 2 (1 × ), CH 4 (28 × ) and N 2 O (265 × ), the relative contribution of the three gases was 74, 19 and 7%, respectively, during the most recent decade ( Table 1 ). Agriculture plays the most significant role in the emission of CH 4 and N 2 O, with enteric fermentation (ruminants) and rice cultivation being the dominant sources of CH 4 , and the increasing use of fertilizer the dominant cause of emissions of N 2 O. Emissions from both gases have increased by 1.6% per year from 1961 to 2010 (ref. 8 ). Together they are responsible for emitting 1.5 PgC per year (5.5 PgCO 2 -eq) or 12% of the total GHG emissions (12.9 PgC per year, 47.3 PgCO 2 -eq; Table 1 ). Thus, agriculture is the second most important source of GHGs after the combustion of fossil fuels. The third largest emission source originates from land-use change ( Fig. 2 ). Given that most of the land-use change is driven by the expansion of cropland and rangelands, food production is currently responsible directly and indirectly for about 20% of anthropogenic GHG emissions. In this context, photosynthesis (CO 2 uptake) and respiration (CO 2 release) in agricultural lands are both large fluxes, but the net exchange is estimated to be a very small sink and statistically indistinguishable from zero at the global scale [9] . To understand the significance of the non-CO 2 emissions, CH 4 and N 2 O emissions counterbalance about 90% of the biological CO 2 sink in continental Europe [10] and 73% of the CO 2 sink in North America [11] . At the global scale, the annual CO 2 -eq flux of anthropogenic CH 4 +N 2 O emissions is larger than the terrestrial net CO 2 sink ( Fig. 2 ). Achieving climate stabilization will require reductions in emissions of the three main greenhouses CO 2 , CH 4 and N 2 O, and the enhancement of the CO 2 sinks to actively remove atmospheric CO 2 . Available types of land-based biological activities include the management of carbon sources and sinks (avoid loss of carbon sinks, increase carbon sinks and decrease GHG emissions) and the replacement of fossil fuels with sustainably produced bioenergy ( Table 2 ). Here we discuss activities available at present with large potentials for climate mitigation underpinned by a high degree of environmental sustainability. This includes a food-first approach, water and soil conservation, avoiding deforestation and conserving biodiversity. We also minimize the contribution of activities with a risk of reversal, that is, the intentional or unintentional release of CO 2 back to the atmosphere, such as afforestation in drought or fire-prone regions. Table 2 Land-based biological climate mitigation activities. Full size table Management of GHG sources and sinks Avoidance of emissions from deforestation and forest degradation is one of the most immediate and largest opportunities available for mitigating climate change. Deforestation is the harvest or burning of forests with the aim to change the land use, for example, to agriculture or urbanization. The rate of forest conversion into other land uses was 13 Mha per year for the period 2000–2010 (ref. 12 ) driving a deforestation gross emission flux of 2.8±0.5 PgC per year (net emissions including forest regrowth are 0.9±0.5 PgC per year) [2] , [13] ( Table 1 ; Fig. 2 ). This flux makes deforestation a major component of the global carbon cycle with 70% of the emissions coming from land-use change in the tropics. These figures illustrate the large mitigation potential in the tropics, but also the equally large challenge to reduce deforestation under the pressure of increasing human population and demand for food and fodder. An initiative of the United Nations Framework Convention on Climate Change is attempting to create a financial value for carbon in forests, providing incentives for less-developing countries to reduce emissions from deforestation and forest degradation, the REDD initiative [14] . Maintaining forests in the tropics would also maintain active carbon sinks, which are estimated to be about 1.2±0.4 PgC per year in established forests (that is, not affected by land-use change) during 2000–2007 (ref. 13 ). One estimate also shows that the forgone carbon sink due to historical and predicted future land-use change will lead to an additional 95 PgC increase in atmospheric CO 2 by 2100, equivalent to an excess of 45 parts per million, p.p.m. (an increase >10% of present atmospheric levels) [15] . In addition, temporary carbon sinks of 1.7±0.5 PgC per year are estimated to come from regrowing tropical forests after abandonment of agricultural land for 2000–2007 (ref. 13 ; Fig. 2 ). Thus, adding the protection of forest regrowth in the context of REDD would greatly extend the mitigation potential available. Beyond benefits in the GHG balance, avoided deforestation in the tropics has additional climate-cooling effects mainly via the cycling of water not considered in current climate policies. Larger amounts of water return to the atmosphere through transpiration and canopy evaporation, which in turn supports the production of convective clouds and rainfall, both of which have cooling effects [16] , [17] . Outside of the tropics, afforestation and forest regrowth on abandoned agricultural land has increased the carbon sinks of North America [18] , Europe [19] and China [20] over the past century. Therefore, enabling abandoned land to regrow forests will continue to enhance the terrestrial sink, although at a significantly declining rate in the future as less fertile land is being abandoned and new forests reach maturity [21] or are harvested. Further sink enhancement is possible through large-scale afforestation programs, particularly those with highly productive eucalyptus, poplar, pine, spruce and Douglas fir species [22] , [23] . However, some of the forest gains in developed countries have been achieved by increasing the fraction of food and wood products imported from developing countries, leading to reduced forest cover and carbon sinks there [24] . Thus, the long-term carbon sequestration potential of this option is limited, particularly in areas not previously forested or if the plantations are not associated with the production of bioenergy (see next section) or wood products. Tree plantations in the extensive semi-arid regions reclaimed from low-production pasture systems are unlikely to be long-term permanent carbon stocks, as they are subject to large climatic inter-annual variability, including drought and fire that release carbon back into the atmosphere. The Intergovernmental Panel on Climate Change (IPCC) has developed a number of concentration and emission scenarios, which effectively describe possible climate futures based on a wide range of socioeconomic scenarios. These so-called Representative Concentration Pathways, RCPs [25] , [26] , support the potential for strong reductions in emissions from land-use change averaging a decline of 80% of present land-use change emissions from 2005 to 2100, with the fastest changes occurring during the first part of the century. Taking net emissions from land-use change in the tropics alone of 1.1 PgC per year (2000–2007) [13] , and assuming a linear trend in emission reductions, we estimate cumulative avoided emissions of 10–22 PgC (50–90%) for the period 2014–2050. These estimates are supported by the steady decrease in emissions from land-use change since 2000 (refs 2 , 25 ), largely due to the slowdown in forest loss from 16 Mha per year during the 1990s to 13 Mha per year during the 2000s (ref. 12 ). At present, pressure remains high to continue making more land available for multiple uses, indicating the need for new legal and economic instruments to maintain recent favourable trends in the future [14] , even though political change may reverse this trend. Both avoided deforestation and reforestation projects require some level of continuous management in perpetuity to reduce the possible impacts of disturbances and associated risk of carbon sequestration reversal [27] , [28] . Insect damage and fires resulting from winter warming trends in Canadian forests are responsible for a historical switch from a net sink to a neutral balance [29] . Recent unprecedented droughts in Amazonia, Southeast Asia and the United States have provided evidence of the high vulnerability of biomass and peat [30] , [31] . Large portions of the world’s most carbon-dense forests found in Australia [32] were burnt in the same year, as the recognition of their extraordinary stock size was published. Such vulnerabilities can be, at best, partially managed through forestry practices including thinning, reducing undergrowth and active fire-risk management, which are linked to a sustainable use of biomass [33] , [34] . The risk of reversal suggests that a cautious approach to large-scale carbon farming projects is necessary. Improved agricultural practices provides additional opportunities for emission reductions with no competition for land or biomass. The focus on technologies that reduce CH 4 and N 2 O emissions brings the added value of no risk for reversal (that is, avoided emissions are permanent). On the basis of the activities responsible for the largest contributions of CH 4 and N 2 O to warming potential, significant mitigation activities include improved quality feed for livestock and manure management, improved regulation of flooding regimes in rice paddies with drainage in the middle of the growing season, reduced burning of agricultural residues and improved timing and precision delivery of N fertilizer ( Table 2 ). The technical potential for agriculture to reduce CH 4 and N 2 O is high and largely driven by the economic valuing of emission reductions. Given the lack of current incentives worldwide, we adopt a lower mean of 0.21 PgC of CO 2 -eq per year by 2030 based on available field studies and modelling for up to US$20 per ton CO 2 -eq (ref. 35 ). This value equates to cumulative avoided emissions of 8 PgC-CO 2 -eq by 2050. Restoration of organic soils has large potential, but remains an expensive undertaking [35] . The rebuilding of depleted soil carbon stocks in degraded crop and pasture lands [9] has a large theoretical potential. They cover over a third of the global ice-free land, particularly in semi-arid regions of Africa, Australia, China and South America. However, carbon gains can be subject to reversibility through drought and fire. On the basis of an optimistic low carbon pricing applied globally [9] , we assess a feasible mitigation potential of a cumulative 8 PgC by 2050. Additional climate mitigation opportunities exist from the demand side of agriculture, including changes in diets and reduced waste and losses in the supply chain [4] , [35] . Bioenergy production The long-term permanence of carbon stocks, which is a concern in avoided deforestation and afforestation activities, makes bioenergy production attractive because it could rely on shorter rotation cropping and harvest of residues ( Table 2 ). The capacity of bioenergy to provide increased energy security for some countries is in no doubt, but the magnitude of the net climate benefits, the potential competition for other land uses and the long-term sustainability of large-scale biomass production need careful consideration. The current (first)-generation of biofuels use food crops such as sugarcane, corn, sugar beet and sweet sorghum for bioethanol; rapeseed, soybean, oil palm and Jatropha are used for biodiesel. The GHG life cycle analyses of these biofuel systems, when compared with their equivalent fossil fuel systems, show ranges of avoided GHG emission from more than 60% for sugarcane in Brazil and wood-based systems to less than 30% reductions for some rapeseed-biodiesel systems in Europe and corn–ethanol in the USA [36] , [37] , [38] . For the latter two systems, new evidence suggests that full emission analysis, including the direct and indirect effects of the potent GHG N 2 O associated with N fertilization, results in highly reduced and, in some cases, no climate benefit ( Box 1 ). Ethanol based on sugarcane crops that do not replace native ecosystems, do not burn residues and return nutrients to the soil to minimize the use of chemical N fertilizer presently has the largest potential for climate mitigation. Many of the current (first)-generation biofuels do not yield net GHG emission savings if their establishment requires the transformation of native ecosystems [39] , [40] , [41] , [42] . This is because emissions from land-use change, which are usually kept separate from life cycle analyses or which are not accounted for, require biofuel systems to accrete GHG reductions for many years before breaking even with the emissions incurred from the initial land transformation (commonly referred to as carbon debt). Repayment of this carbon debt has been estimated to be 17 years for a sugarcane–ethanol system in Brazil replacing woody cerrado, 93 years for a corn–ethanol system replacing grasslands in central USA and 840 years for a biodiesel–oil palm system replacing rainforest on deep peatland in Southeast Asia [39] . Lignocellulosic crops (that is, second-generation biofuels) such as Miscanthus , poplar and switchgrass ( Panicum virgatum ) have more favourable GHG savings potential than many food-based crops [43] , [44] , and therefore offer a more attractive mitigation option ( Fig. 3 ). Particularly, low-management input woody and grassy perennial systems on degraded lands and on lands not suitable for food crops are regions to further promote biomass production. This includes monoculture crops such as Miscanthus or switchgrass and mixtures of native grasses that are best suited to impoverished soils and that have the capacity to improve soil condition and carbon content [45] , [46] , [47] . Sustainable deployment of these activities requires attention to the potential of high biodiversity value of some marginal lands. 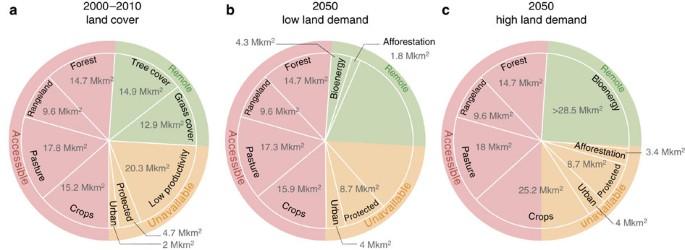Figure 3: Current land cover and future land demands. Land cover and land demands as they relate to use and suitability for human appropriation. The land biosphere (excluding bare lands, Antarctica and Greenland) of 112 km2is divided into three land categories (colours): available (salmon), indicating accessible and suitable land for human appropriation (all already under different levels of appropriation at present); unavailable (orange), indicating non-availability of land (for example, conservation land) or unsuitable land because of very low plant productivity; and remote (green), indicating land too far from human settlements to be managed by human activities (for example, remote tundra). (a) 2000–2010 distribution of land cover; (b) low range of land demands for multiple purposes by 2050; (c) high range of land demands by 2050. Sources: (a) all land cover shown in the figure, except urban, are taken from ref.79; urban estimates are taken from ref.80. (b) Crops requiring large increases in yields and cropping intensity81; pasture from the mean decline of 3% from IPCC scenarios (RCP2.6, 3.5 and 6.0); rangeland and forests79; bioenergy using abandoned land only63; afforestation based on 2005–2010 trends of 5 Mha per year12to 2050; protected areas80; urban estimates to 2030 (ref.55) extended to 2050. (c) Crops based on current trends of intensification and extensification53; pasture based on 1% increase in IPCC scenario RCP8.5 (ref.25); rangeland and forests79; bioenergy up to 36 km2(ref.82); afforestation to achieve 1.5 pg per year by 205061; protected areas80; urban estimates to 2030 (ref.55) extended to 2050. Figure 3: Current land cover and future land demands. Land cover and land demands as they relate to use and suitability for human appropriation. The land biosphere (excluding bare lands, Antarctica and Greenland) of 112 km 2 is divided into three land categories (colours): available (salmon), indicating accessible and suitable land for human appropriation (all already under different levels of appropriation at present); unavailable (orange), indicating non-availability of land (for example, conservation land) or unsuitable land because of very low plant productivity; and remote (green), indicating land too far from human settlements to be managed by human activities (for example, remote tundra). ( a ) 2000–2010 distribution of land cover; ( b ) low range of land demands for multiple purposes by 2050; ( c ) high range of land demands by 2050. Sources: ( a ) all land cover shown in the figure, except urban, are taken from ref. 79 ; urban estimates are taken from ref. 80 . ( b ) Crops requiring large increases in yields and cropping intensity [81] ; pasture from the mean decline of 3% from IPCC scenarios (RCP2.6, 3.5 and 6.0); rangeland and forests [79] ; bioenergy using abandoned land only [63] ; afforestation based on 2005–2010 trends of 5 Mha per year [12] to 2050; protected areas [80] ; urban estimates to 2030 (ref. 55 ) extended to 2050. ( c ) Crops based on current trends of intensification and extensification [53] ; pasture based on 1% increase in IPCC scenario RCP8.5 (ref. 25 ); rangeland and forests [79] ; bioenergy up to 36 km 2 (ref. 82 ); afforestation to achieve 1.5 pg per year by 2050 [61] ; protected areas [80] ; urban estimates to 2030 (ref. 55 ) extended to 2050. Full size image Additional lignocellulosic feedstock can come from agriculture crop and wood residues. They offer larger climate benefits than food crops, do not necessarily require new land, and if harvested sustainable, they can offer an effective climate mitigation activity. The overall potential of residues as a source of biomass, however, is very limited, as continued inputs of agricultural and forest residues into the soil are required to maintain soil fertility [48] , [49] ( Table 3 ). Table 3 Sustainable potentials of global primary energy from bioenergy by 2050. Full size table Table 2 shows global estimates of the technical potential of primary energy from bioenergy that could be achieved by 2050, ranging from 26 to 161 EJ per year with associated land demands between 133 and 990 Mha. All estimates include various levels of environmental sustainability constraints, but some estimates do not account for the full GHG balance including fertilizer production and use. They have large reliance on crop and forestry residues, they allow for further deforestation or they are not constrained by water and other resource limitations. Here we adopt the minimum values reported in Table 2 as the bioenergy potential that meets a comprehensive set of criteria for environmental sustainability. It suggests a global potential of 26–64 EJ per year of primary energy by 2050. The climate benefits, however, could increase significantly if bioenergy systems are coupled to carbon capture and storage, as it is being extensively modelled in the design of energy portfolios to achieve climate stabilization by 2100 ( Box 2 ). Box 1: N 2 O emissions and the intensification of biomass production. The nitrogen (N) cycle is intrinsically coupled to the carbon cycle because the physiology of organisms is regulated by proteins, all of which contain N. Thus, enhancement of biomass production for the purpose of increasing food and feedstock for bioenergy production requires inputs of N via chemical or organic fertilization or biological N 2 fixation. An intensification of the N cycle will lead to an increase in the emission of nitrous oxide (N 2 O). N 2 O emissions originate from the two main microbial reactions, nitrification (oxidation of ammonium, NH 4 + , to nitrite, NO 3 − ) and de-nitrification (reduction of nitrate). During nitrification, the reduced form of N, mainly NH 4 , may enter the cell while NO 3 is being formed, alternatively, NO 3 is taken up and denitrifies to N 2 . In both reactions, the intermediate products NO and N 2 O may leak out of the cell. N 2 O is 265 times more powerful a GHG than CO 2 on a time horizon of 100 years [92] . Its atmospheric concentration has increased by 21% since pre-industrial times, and it is now the third most important well-mixed GHG contributing to human-driven climate change after CO 2 and CH 4 (ref. 25 ). N 2 O is also a dominant ozone-depleting substance. N 2 O emissions from the Green Revolution over the past half-century, where global N fertilizer use increased by eightfold [52] , led to the rapid growth of atmospheric N 2 O (ref. 25 ). There are concerns that continued intensification of agriculture, and the rapid expansion of highly productive bioenergy crops will further increase the atmospheric burden of anthropogenic N 2 O and reduce the climate benefits of bioenergy [37] . The N emission conversion factor (to N 2 O) is the fraction of N 2 O-N that is emitted for a given amount of N fertilizer applied or biologically fixed N. The IPCC Guidelines for National Greenhouse Gas Inventories [93] has set this quantity, as a default value, to 1% for direct emissions and to 0.34–0.40% for indirect emissions (emissions from volatilization, leaching and runoff). However, more recent estimates show that food-based high-input biofuel crops have N conversion factors between 2 and 7% for sugarcane [85] , rapeseed [86] and corn [94] . Two recent global estimates of the N conversion factor range from 2.5 to 5% (refs 95 , 96 ), which is about 2–3 times higher than the ones used in the IPCC Guidelines [93] . On the basis of these new global estimates, current bioenergy cropping for diesel–rapeseed and ethanol–corn would provide little climate benefits or even net warming, while other crops would have climate benefits below what has been reported. Managing N 2 O emissions presents a significant mitigation opportunity given that for every 100 units of N applied to the crop system, only 17 make their way into the food we eat [97] . One such opportunity is to improve N management through fertilizer applications that are synchronized with plant development to minimize N 2 O emissions from excess N use. The largest mitigation potentials are in countries with the highest excessive fertilizer use such as China, Northern India, USA and Western Europe [52] , while developing countries with lower yields present the biggest opportunities for technology transfer on nutrient management. Box 2: Bioenergy with carbon capture and storage. Bioenergy with Carbon Capture and Storage (BECCS) is a mitigation technology that combines biomass use with geological carbon capture and storage to produce negative CO 2 emissions. Atmospheric CO 2 is effectively captured by plants during photosynthesis and fixed into biomass, which is then used for bioenergy production. The CO 2 emitted during this process is subsequently captured and sequestered in geological reservoirs, most commonly saline aquifers. This chain of processes, including the substitution of fossil fuel use with the bioenergy produced and the subsequent crop regrowth or replanting, creates a net carbon sink, or net negative emissions, in addition to a valuable source of energy. Biomass can be combusted, fermented, digested or gasified leading to different energy products such as heat, electricity, methane and synthetic biofuels. Interestingly, BECCS can be applied to diverse industrial sectors such as combustion biomass power plants, combined heat and power plants, pulp industry, biomass gasification and ethanol fermentation [98] . The coupling of non-energy biorefining processes can lead to additional benefits towards the financial attractiveness of BECCS, such as the production of green chemicals, bioplastics and plastic resins. The importance of BECCS as a negative emission technology comes from the widening gap between requirements for safer climate-stabilization levels (for example, keeping global temperature under 2 °C above pre-industrial levels) and current growth rates of fossil fuel emissions. Most global assessments require the assumption of negative emission technologies to meet the mitigation requirements of low temperature stabilization scenarios [65] , [99] . Significantly, two-thirds of the Earth system models used in the latest IPCC report [50] require GHG emissions to approach zero by the second part of this century and a net removal of atmospheric CO 2 thereafter to stabilize global temperatures under 2 °C (refs 25 , 54 ). Even in models and scenarios where net global negative emissions might not be required, BECCS is assumed to compensate emissions from sectors too difficult to mitigate, such as agriculture and aviation [65] . Biomass-based negative emission technologies face the same challenges as other biospheric mitigation options, namely, the deployment of large-scale sustainable biomass-production systems and efficient transport systems to collect biomass. BECCS also requires the existence of carbon prices high enough to make the expensive investment in carbon capture and storage facilities financially viable. Such prices are unlikely to be realized until later in this century at best, particularly if strong mitigation action is globally pursued. Global mitigation potentials and land requirements The sustainable potential of land-based biological mitigation requires us to solve the quandary of how to meet the demands for climate protection, energy security, food security and biodiversity conservation, at both global and regional scales. Specifically, how we can (1) increase food production to feed a growing and more affluent population, (2) increase carbon sinks to reduce excess atmospheric CO 2 , (3) produce energy from biomass to increase energy security and (4) reduce human encroachment into native ecosystems. Simultaneously, there is a further need to reduce anthropogenic GHG emissions from the combined human activity to near zero if climate stabilization is to be achieved [50] . A conceptual baseline for sustainable carbon sequestration potential can be obtained by considering the carbon gains achievable from returning the historical cumulative emissions from land-use change back into biospheric carbon pools. Such a scenario would involve regrowing native vegetation on lands from which native vegetation has been removed by human activity. This fictional scenario, which leaves no room for food production or any other uses, would lead to a reduction of 40–70 p.p.m. of atmospheric CO 2 by the end of this century [51] . This is equivalent to 16–28% of the emission reductions required to stabilize the climate under 2 °C by 2100 (RCP2.6) compared with a high carbon intensity scenario (RCP8.5). Contrasting with this hypothetical scenario, land requirements from different sectors of society are multiple, large and interconnected in ways that make the partition of land uses a major challenge. Figure 3 illustrates the current land cover and the range of future land demands under different scenarios and expectations for specific uses. Current crops and pastures have already appropriated 14 and 30% of the ice-free land, respectively [52] . This area would need to increase by over 1,000 Mha to feed 9 billion people [53] under current trends of intensification and extensification, occupying together with current pastures close to 50% of all lands. Three of the four new IPCC scenarios (RCPs) require increased cropland area to feed the world population by 2100 at the expenses of forests and available pasture land (the latter due to the intensification of the livestock sector) [54] . It is also estimated that rapid global urbanization will take an additional 120 Mha of land by 2030 alone to accommodate 1.3 billion new urbanites [55] . A large fraction of this expansion will be on fertile plains of high agricultural value, with further erosion of coastal plains due to sea level rise [56] . Future projections of bioenergy potential and their land requirements are also large. Estimates of the Global Energy Assessment [57] on global primary bioenergy potential by 2050 range from 32 to 1,271 EJ per year with commensurate requirements for land between 470 and 3,590 Mha (ref. 57 ) ( Fig. 3 ). The IPCC narrows the potential between 100 and 300 EJ per year, equivalent to 20–60% of current global primary energy [58] . In comparison, the chemical energy value of all current global biomass use in food, fibre, feed, wood products and traditional wood use is 230 EJ per year [59] . Additional land pressure arises from the identified potentials to sequester 0.2–1.5 PgC per year in new forests and plantations requiring land areas of up to 345 Mha (refs 60 , 61 ), equivalent to increasing the current forested area by 18% ( Fig. 3 ). One study that takes into account the ecological limits of productivity and the need for N and phosphorus to grow new biomass estimates the need of 7 Mha of eucalyptus plantations in highly productive tropical regions or 200 Mha of switchgrass in temperate regions with carbon capture and storage to achieve each a mitigation of 1 PgC per year [62] . The estimates for land demands by 2050 in Fig. 3 come from independent assessments, which neglect the fact that some of the demands aim to use the same land areas, called ‘double counting’. However, these independent assessments illustrate well the large future pressures on land. The high land demand assessment ( Fig. 3c ) requires more land than that existing free of ice or barren soil. Taking the mean value of the low and high demands in Fig. 3b,c , the total future demand, or expectations for potentials to realize, require about 3,000 Mha, 3–7 times an area larger than the land identified as abandoned, marginal or of low productivity under different assumptions (428–1,035 Mha) [63] , [64] . Here we assemble the various mitigation potentials discussed and show that it is feasible to produce cumulative emission avoided and emission reductions of up to 26–38 PgC-CO 2 -eq by 2050 with no requirement for additional land (see section Management of GHG sources and sinks). This mitigation consists of 10–22 PgC from the reduction of current land-use change emissions dominated by avoided deforestation and degradation, most of it occurring in tropical regions, up to 16 PgC-CO 2 -eq from improved agricultural practices, half from reduced CH 4 and N 2 O emissions and the other half from improved/restored soil carbon. Although in some instances current trends are consistent with achieving some mitigation, new legal and economic instruments are required to achieve the full potentials and to achieve larger ones [35] . We compare the requirements to stay under 2 °C above pre-industrial by 2080–2100 (RCP2.6, 0.9–2.3 °C above pre-industrial) with the future carbon trajectories of a low and a high carbon intensity scenarios as references to explore the entire spectrum of possible mitigation: RCP4.5 (1.7–3.2 °C) and RCP8.5 (3.2–5.4 °C) [26] . The cumulative mitigation required by 2050 ranges between 170 PgC-CO 2 -eq (625 PgCO 2 -eq) and 397 PgC-CO 2 -eq (1,456 PgCO 2 -eq). Thus, avoided deforestation emissions and reduced emissions from agriculture can contribute from between 6 and 22% of the total mitigation required. Since early 2000, trends in carbon emissions have been tracking the most carbon intense scenario (RCP8.5) [2] , [65] , which, if unchanged, would result in the lower of estimated contributions of land-based mitigation to climate stabilization. Additional mitigation is available from the sustainable production of bioenergy largely in abandoned agricultural lands and therefore with the lowest risk for competition with other land uses (see section Bioenergy production). This could displace the use of fossil fuel energies by 26 and 64 EJ per year, equivalent to 3–8% of the total primary energy by 2050, assuming a 60% increase in energy consumption (about 800 EJ, consistent with intermediate IPCC scenarios). At the national level, these contributions can be significantly higher for tropical countries with large opportunities for avoided deforestation and biomass production, but it will be lower for countries elsewhere with high rates of fossil fuel consumption. The success of three major components of future research and development, namely, (1) sustainable intensification of land, (2) algae-based biofuels and (3) bio-inspired catalytic systems, can potentially increase the current contribution of biologically based mitigation in significant ways. Sustainable intensification of land One of the biggest opportunities for land-based mitigation activities relies on the development of a new model for sustainable intensification of land, which can accommodate growing demands on biomass production for food, bioenergy, conservation and carbon sinks. Intensification opportunities exist in three key areas: (1) yield intensification, which is the increase in crop production per area. This needs to begin with the closing of the so-called yield gap globally, which is the yield difference between lower-yielding production systems and the highest yields that can be achieved under best practices in similar environmental conditions. Closing the yield gap can increase global production without the requirement for additional land by 45–70%, leading to more than 2 billion tons of additional food and feed crops [52] , [53] , [66] . Higher yields can also be achieved by better selection of species and varieties. (2) Temporal intensification, which requires an increase in the number of crops per year, aided by a broader crop diversification including crops for food, feed and bioenergy [67] and (3) spatial intensification, which pursues land optimization and the implementation of best practices in addressing trade-off among multiple competing land uses. It calls for an integrated and comprehensive approach to managing land systems covering all production and conservation uses. This approach poses large challenges for institutional governance and land property rights, but can yield big environmental and climate benefits. Critical to the sustainable intensification of biomass production in components (1) and (2) is improving N management to minimize N 2 O emissions from excess N, and the use of N-fixing cover crops to increase soil N. It is possible to close the global yield gaps on major cereals to within 75% of achievable yields with current amounts of N and phosphate use [66] . Other environmental impacts such as groundwater pollution can also be reduced through higher precision input management. Algae-based biofuels The success of microalgae-production systems is key to developing the third generation of biofuels. Algae are able to accumulate large quantities of lipids for biodiesel production, with little or no requirements for productive land. They could provide an alternative to one of the most intractable problems of large-scale deployment of biomass production [68] . To date, microalgae–bioenergy systems have not achieved the required benefits in GHG savings when compared with fossil fuel-based biodiesel, nor have they achieved acceptable levels of environmental sustainability [68] , [69] . The largest energy requirements usually come from the use of nutrients required to grow algae, particularly N [70] , while the biggest challenge in environmental sustainability comes from the large requirements for water and nutrients. These include the use of 3 to >3,500 litres of freshwater for each litre of algae–biofuel produced, and 44–107% and 20–51% of today’s United States’ use of N and phosphorus, respectively, to produce just 5% of the current US fuel market. Furthermore, large use of antibiotics to keep algae cultures disease free remains an unresolved issue. To address these challenges, future research directions include: (1) ways to reduce the nutrient demand by recycling wastewaters containing significant quantities of nitrate and phosphates; (2) the production of new algal strains that have higher growth rates and lipid accumulation and higher tolerance to contaminants; and (3) new designs of open and closed bioreactors to culture algae with smaller energy and antibiotics requirements. The prospects for biorefining diversification for the pharmacy and food industries would further help in designing cost-benefit processes that have more favourable GHG balance and sustainability outcomes [68] , [69] , [71] . The development of aviation fuels is a unique opportunity niche for microalgae bioenergy given that other renewable energies are less suitable to provide fuels with the high-energy content that is required to power aeroplanes. Bio-inspired catalytic systems Dihydrogen (H 2 ) is a clean, renewable energy carrier, the oxidation of which produces heat and water as the only products [72] . H 2 is also central to many industrial processes such as the production of N fertilizer, and in combination with the use of H 2 to reduce CO 2 to CO, gas mixtures would be suitable for the production of carbon-based fuels like methanol [73] (with the co-benefit of capturing CO 2 emitted by other processes). We take dihydrogen gas as a centre point and describe a number of possible bio-inspired catalytic systems that could generate clean energy and industrial products. 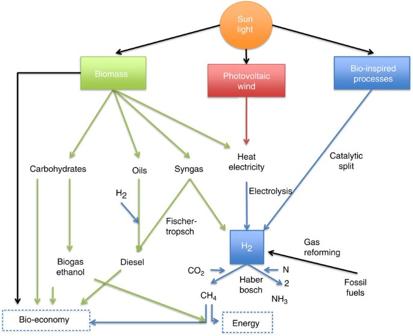Figure 4: Multiple uses of sunlight for producing energy products. There are three main energy-production systems: biomass (green), direct use through photovoltaic and wind (red) and bio-inspired processes (blue). Each system produces a unique set of energy products for different applications, such as biomass to carbohydrates, oil, gases and heat. Because these processes operate with variable time-dependent output and efficiency (for example, wind and photovoltaic depend on weather conditions), a common chemical platform integrates the multiple production pathways. The production of H2gas (blue) serves this function, even though the technical handling of H2remains difficult due to its low density, high diffusivity and chemically corrosiveness. Figure 4 shows how sunlight has been used or could be used in the future. Biomass can be the basis for various liquid fuels (ethanol and biogas from carbohydrates and biodiesel from lipids), or as basis for chemical industries after fermentation into various chemical processes. Alternatively, lignocellulosic biomass can be gasified into ‘syngas’, a mixture of CO and H 2 , which could either be catalysed via the Fischer–Tropsch process again into ‘synthetic diesel’ or purified into H 2 as a base product for chemistry and energy [74] , [75] , or converted to methanol [73] . Heat and electricity can be generated from biomass to produce H 2 via electrolysis. New discoveries on biocatalysis of CO 2 hydrogenation (CO 2 +H 2 ) by bacteria can produce storage fuels (for example, formic acid) chemically equivalent of H 2 and used as fuel cells [76] . Figure 4: Multiple uses of sunlight for producing energy products. There are three main energy-production systems: biomass (green), direct use through photovoltaic and wind (red) and bio-inspired processes (blue). Each system produces a unique set of energy products for different applications, such as biomass to carbohydrates, oil, gases and heat. Because these processes operate with variable time-dependent output and efficiency (for example, wind and photovoltaic depend on weather conditions), a common chemical platform integrates the multiple production pathways. The production of H 2 gas (blue) serves this function, even though the technical handling of H 2 remains difficult due to its low density, high diffusivity and chemically corrosiveness. Full size image Putting H 2 as a central energy carrier combines and mixes several energy sources and makes them exchangeable. In this context, a novel emerging process becomes important, the catalytic splitting of water through bio-inspired processes (that is, artificial photosynthesis). These processes include the isolation of photosynthetic enzymes and their use in artificial systems or biocatalytic and photoelectrolytic systems, which would split water based on solar energy and collect the electron during formation of dihydrogen [74] . In these cases, either natural proteins or novel catalyzers resembling the natural photosystem and the hydrogenase are the active centres for H 2 production. These bio-inspired artificial systems are at early stages of research and development, but if successful would reduce pressure on land [71] . Future challenges include increasing system efficiency and developing new chemical reactions under conditions of variable inputs and reactor conditions. Currently available land-based biological mitigation has and will have an important role in achieving climate stabilization, largely from reduced emissions from land use and land-use change and from the substitution of fossil fuels with sustainably produced bioenergy. With current technologies, the potential for land mitigation is significant, but relatively small when compared with the overall mitigation requirements for climate stabilization. Future growth in the contribution of bio-based mitigation will depend on the success of developing systems that minimize the requirements for additional land and nutrients, and contribute to the sustainable intensification of land. Sustainable intensification of land requires a new and unprecedented integrated research effort. This needs to contribute to precision ecosystem-level management of inputs and resources, while developing a comprehensive framework for regional optimization of land uses, including conservation. Advancements are required in both technological innovation and large interdisciplinary collaboration such as the one of Future Earth of the International Council for Science. Other research and technological innovation can lead to increasing photosynthetic potentials in non-land-based systems, and the development of bio-inspired technology will remain a research frontier for years to come with as yet unproven potentials to contribute to climate stabilization. How to cite this article: Canadell, J. G. and Schulze, E. D. Global potential of biospheric carbon management for climate mitigation. Nat. Commun. 5:5282 doi: 10.1038/ncomms6282 (2014).